DJ-1 promotes angiogenesis and osteogenesis by activating FGF receptor-1 signaling Communication between osteoblasts and endothelial cells is essential for bone fracture repair, but the molecular identities of such communicating factors are not well defined. Here we identify DJ-1 as a novel mediator of the cross-talk between osteoblasts and endothelial cells through an unbiased screening of molecules secreted from human mesenchymal stem cells during osteogenesis. We show that DJ-1 stimulates the differentiation of human mesenchymal stem cells to osteoblasts and that DJ-1 induces angiogenesis in endothelial cells through activation of fibroblast growth factor receptor-1 signalling. In a rodent model of bone fracture repair, extracellular application of DJ-1 enhances bone regeneration in vivo by stimulating the formation of blood vessels and new bones. Both these effects are blocked by antagonizing fibroblast growth factor receptor-1 signalling. These findings uncover previously undefined extracellular roles of DJ-1 to promote angiogenesis and osteogenesis, suggesting DJ-1 may have therapeutic potential to stimulate bone regeneration. Angiogenesis, the formation of new vascular networks, is an essential process for wound healing and is subject to multiple layers of regulation during the migration and proliferation of endothelial cells and their subsequent differentiation into mature blood vessels [1] . These processes are mediated by components of the extracellular matrix (ECM), cytokines and growth factors, such as vascular endothelial growth factor (VEGF) and fibroblast growth factors (FGFs). Among them, FGF-2 is known to stimulate angiogenesis in vivo [2] and promote endothelial cell proliferation, chemotaxis and tube formation in vitro [1] , [3] . In endothelial cells, FGF-2 exerts its biological effects mainly by activating fibroblast growth factor receptor-1 (FGFR-1) [4] , [5] , [6] , [7] , which is a member of the tyrosine kinase receptor family [8] , [9] , [10] . FGF-2 also induces VEGF expression in endothelial cells through autocrine and paracrine mechanisms [11] . Bone fracture healing is a complex process mediated by multiple factors and is known to proceed through definable temporal and spatial sequences. In particular, cell-to-cell communication between diverse cell-types, such as endothelial cells, osteoblasts, osteoclasts and fibroblasts, is vital to the healing process [12] , [13] , [14] . Impaired bone healing is associated with a reduction in vascular supply and limited nutrient availability at the site of injury, suggesting that an impaired angiogenic response is a major cause for this pathology [13] , [14] , [15] , [16] , [17] . Accordingly, angiogenic factors, such as VEGF and FGFs, which are upregulated during the healing process, are thought to have important roles in repairing bone fracture [18] , [19] . Several reports have demonstrated an intricate interplay between bone-forming osteoblasts and vessel-forming endothelial cells, consistent with their physical proximity during bone formation [18] , [20] . In particular, osteoblasts secrete angiogenic (such as VEGF) and osteogenic (such as insulin-like growth factor-I) factors, which mediate the cross-talk between osteoblasts and endothelial cells [21] . Given that cell-to-cell communication has a critical part during the healing process, we have searched for additional angiogenic factors that are specifically secreted from osteoblasts. By applying a systematic proteomic approach, here we identify DJ-1 as a novel angiogenic factor secreted from human mesenchymal stem cells (hMSCs) during osteogenesis. Human DJ-1, which is a 189-amino acid protein encoded by PARK7 , is ubiquitously expressed in various human tissues [22] . Mutations in the DJ-1 gene are known to cause familial Parkinson’s Disease [23] and DJ-1 has been suggested to have chaperone-like [24] and pro-survival activities [25] , [26] . In addition to its intracellular functions, several studies have reported that DJ-1 is secreted into the extracellular regions [27] , [28] , but the extracellular role of DJ-1 has remained enigmatic. In this study, we have found that DJ-1 mediates the cross-talk between osteoblasts and endothelial cells. We provide evidence that DJ-1 promotes osteogenesis and induces angiogenesis through the activation of FGFR-1 signalling both in vitro and in vivo. Moreover, we show that in a rodent model of bone fracture repair, application of DJ-1 directly to the injured site markedly enhances bone regeneration by stimulating the formation of blood vessels and new bones. Consistent with the role of DJ-1 in osteogenesis, mineralization of osteoblasts and bone regeneration processes are impaired in DJ-1 -knockout mice. Taken together, these results reveal previously undefined extracellular functions for DJ-1 as an angiogenic and an osteogenic factor, suggesting a therapeutic potential of DJ-1 in bone fracture healing and bone regeneration. Osteoblast conditioned medium enhances endothelial cell migration To identify previously unidentified secretory molecules that promote angiogenesis during osteogenesis, we collected conditioned medium (CM) from undifferentiated hMSCs or differentiated osteoblasts ( Fig. 1a ). CM was collected at 10th day after the induction of osteogenesis because at this time we were able to detect substantial mineralization of ECM, characteristic of mature osteoblasts. Differentiation of hMSCs into osteoblasts was confirmed by alizarin red S staining to detect mineral accumulation in the ECM ( Supplementary Fig. S1a,b ). Quantitative reverse transcription-PCR was also performed to measure the levels of osteogenic markers, such as alkaline phosphatase (ALP), runt-related transcription factor 2 (Runx2), bone sialoprotein (BSP) and osteocalcin (OCN) ( Supplementary Fig. S1c ). By employing a modified Boyden chamber assay [29] , we then examined if the CM from undifferentiated hMSCs or osteoblasts had any effects on the migration of immortalized human umbilical vein endothelium cells (iHUVECs), a property which is related to angiogenesis. As compared with the CM collected from undifferentiated hMSCs, osteoblast CM significantly enhanced the migration of iHUVECs in a concentration-dependent manner ( Fig. 1b ). On the other hand, osteoblast CM lacking VEGF was sufficient to induce the migration of iHUVECs and osteoblast differentiation ( Supplementary Fig. S2 ). 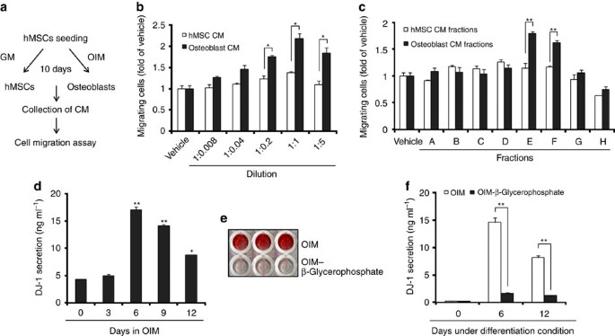Figure 1: Experimental strategy and DJ-1secretion during osteogenesis of hMSCs. (a) Experimental strategy for identifying novel angiogenic factors secreted during osteogenesis. After hMSCs were seeded for CM collection, one group was cultured in growth medium (GM) and the other group was cultured in osteogenesis induction medium (OIM). After 10 days, the CM from undifferentiated hMSCs and differentiated osteoblasts were harvested and examined for effects on iHUVEC migration. (b) After concentrating the hMSC and osteoblast CM, CM were applied at varying concentrations as indicated and effects on iHUVEC migration were analysed. After incubation for 6 h, migrating cells were quantified. Migrating cells were expressed as the fold-change in comparison to the vehicle, which contained only the medium. *P<0.05 versus hMSC CM. (c) hMSC and osteoblast CM were separated by reverse-phase high-performance liquid chromatography and fractions were tested for iHUVEC migration-inducing activity. After incubation for 6 h, migrating cells were analysed. Migrating cells were expressed as the fold-change in comparison to the vehicle control. **P<0.01 versus the hMSC CM fractions. (d) The concentration of DJ-1 in the medium (collected from 0 to 12 days after osteogenesis induction) was quantified by enzyme-linked immunosorbent assay. *P<0.05 and **P<0.01 versus day 0. (e) Depletion of β-glycerophosphate from the OIM drastically prevented mineral accumulation of osteoblasts. Alizarin red S staining was performed at 12 days after the induction of osteogenesis. (f) DJ-1 secretion was quantified after treatment with OIM that contains or lacks β-glycerophosphate. **P<0.01 versus OIM treatment.n=3 for all groups. All data are expressed as means±s.e.m. Figure 1: Experimental strategy and DJ-1secretion during osteogenesis of hMSCs. ( a ) Experimental strategy for identifying novel angiogenic factors secreted during osteogenesis. After hMSCs were seeded for CM collection, one group was cultured in growth medium (GM) and the other group was cultured in osteogenesis induction medium (OIM). After 10 days, the CM from undifferentiated hMSCs and differentiated osteoblasts were harvested and examined for effects on iHUVEC migration. ( b ) After concentrating the hMSC and osteoblast CM, CM were applied at varying concentrations as indicated and effects on iHUVEC migration were analysed. After incubation for 6 h, migrating cells were quantified. Migrating cells were expressed as the fold-change in comparison to the vehicle, which contained only the medium. * P <0.05 versus hMSC CM. ( c ) hMSC and osteoblast CM were separated by reverse-phase high-performance liquid chromatography and fractions were tested for iHUVEC migration-inducing activity. After incubation for 6 h, migrating cells were analysed. Migrating cells were expressed as the fold-change in comparison to the vehicle control. ** P <0.01 versus the hMSC CM fractions. ( d ) The concentration of DJ-1 in the medium (collected from 0 to 12 days after osteogenesis induction) was quantified by enzyme-linked immunosorbent assay. * P <0.05 and ** P <0.01 versus day 0. ( e ) Depletion of β-glycerophosphate from the OIM drastically prevented mineral accumulation of osteoblasts. Alizarin red S staining was performed at 12 days after the induction of osteogenesis. ( f ) DJ-1 secretion was quantified after treatment with OIM that contains or lacks β-glycerophosphate. ** P <0.01 versus OIM treatment. n =3 for all groups. All data are expressed as means±s.e.m. Full size image To isolate proteins and/or peptides that induced iHUVEC migration, we then performed reverse-phase high-performance liquid chromatography for CMs from undifferentiated hMSCs and differentiated osteoblasts. A total of 96 fractions from each CM were collected and screened for iHUVECs migration-inducing activity. Initially, 96 fractions from each CM were pooled into eight groups, for example, group A contained fractions from A1 to A12. Among the eight groups, groups E and F from osteoblast CM increased iHUVEC migration as compared with the CM from undifferentiated hMSCs ( Fig. 1c ). DJ-1 is secreted during hMSC osteogenesis To identify the molecule responsible for inducing cell migration, we performed electrospray ionization liquid chromatography-mass spectrometry analysis for fractions E and F (mentioned above) obtained from undifferentiated hMSC CM and differentiated osteoblast CM. Through the mass analysis of groups E and F, we were able to identify about 180 proteins and peptides. The fractions contained osteonectin, a well-known secretory molecule that has an essential role in bone mineralization [30] and angiogenesis [31] , together with several additional proteins that have angiogenic activities, such as macrophage migration inhibitory factor [32] (data not shown). Interestingly, the level of DJ-1, a protein whose extracellular function is unknown to date, was markedly upregulated in the CM from differentiated osteoblasts (4.15-fold increase when quantified by mass analysis) as compared with that from undifferentiated hMSCs. When the amount of DJ-1 secretion was quantified by enzyme-linked immunosorbent assay, we found that DJ-1 secretion was increased in response to the induction of osteogenesis with a peak level detected at 6th day ( Fig. 1d ). As this peak in DJ-1 secretion correlated well with the time when mineralization was initiated, we investigated whether mineralization of osteoblasts is associated with DJ-1 secretion. Indeed, DJ-1 secretion was remarkably suppressed when mineralization of osteoblasts was prevented by depleting β-glycerophosphate from the osteogenesis induction medium ( Fig. 1e ). On the other hand, the gene expression level of DJ-1 did not show a similar aspect with the secretion level of DJ-1 during osteogenesis ( Supplementary Fig. S3 ). Taken together, these results suggest that DJ-1 secretion is upregulated during osteogenesis and mineralization of osteoblasts might regulate the translocation of DJ-1 to the extracellular region. DJ-1 stimulates angiogenesis in vitro and in vivo To investigate the possible role of DJ-1 in endothelial cells, we first examined the activity of recombinant DJ-1 in a migration assay using iHUVECs. Recombinant DJ-1 was purified as previously described [24] and verified ( Supplementary Fig. S4 ). We found that DJ-1-induced iHUVEC migration in a dose-dependent manner ( Fig. 2a ). At the dose which DJ-1 exhibited its maximal effect (10 nM), DJ-1 increased iHUVEC migration about 1.5-fold over the vehicle control, the extent which was comparable to well-known angiogenic factors, such as VEGF (20 ng ml −1 ) and FGF-2 (20 ng ml −1 ). 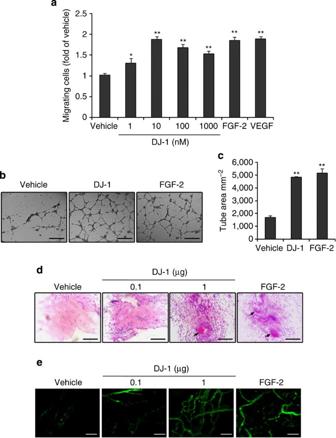Figure 2: DJ-1 functions as an angiogenic factorin vitroandin vivo. (a) DJ-1 induces iHUVEC migration in a dose-dependent manner. Migration-inducing activity of DJ-1 was compared with that of FGF-2 (20 ng ml−1) or VEGF (20 ng ml−1). After incubation for 6 h, migrated cells were fixed, stained and counted in five random fields. Migrating cells were expressed as the fold-change in comparison to the vehicle control. *P<0.05 and **P<0.01 versus the vehicle. (b) iHUVECs were incubated with matrigel in the presence of DJ-1 (10 nM) or FGF-2 (20 ng ml−1). FGF-2 was used as a positive control. Photographs (X50) were taken at 9 h after the treatment. The scale bar represents 400 μm. (c) Quantification of DJ-1-induced capillary tube formation. The tube area was quantified by using Scion image software to measure the tube length of iHUVECs connected to each other in the capillary-like structure. Tube area is presented as the average value from three random fields. **P<0.01 versus the vehicle. (d,e) DJ-1 stimulates angiogenesisin vivo. Matrigel plugs containing vehicle, DJ-1 (0.1 or 1 μg) or FGF-2 (0.1 μg) were subcutaneously injected into mice. After 7 days, the matrigel plugs were extracted, fixed, embedded in paraffin, sectioned at 4 μm and immunostained. (d) Sections of each matrigel plug were stained by H&E and photographed (X200). The arrow shows blood vessels containing red blood cells. The scale bar represents 10 μm. (e) The matrigel plugs were stained with antibody against PECAM (CD31). The scale bar represents 60 μm.n=3 for all groups. All data are expressed as means±s.e.m. Figure 2: DJ-1 functions as an angiogenic factor in vitro and in vivo . ( a ) DJ-1 induces iHUVEC migration in a dose-dependent manner. Migration-inducing activity of DJ-1 was compared with that of FGF-2 (20 ng ml −1 ) or VEGF (20 ng ml −1 ). After incubation for 6 h, migrated cells were fixed, stained and counted in five random fields. Migrating cells were expressed as the fold-change in comparison to the vehicle control. * P <0.05 and ** P <0.01 versus the vehicle. ( b ) iHUVECs were incubated with matrigel in the presence of DJ-1 (10 nM) or FGF-2 (20 ng ml −1 ). FGF-2 was used as a positive control. Photographs (X50) were taken at 9 h after the treatment. The scale bar represents 400 μm. ( c ) Quantification of DJ-1-induced capillary tube formation. The tube area was quantified by using Scion image software to measure the tube length of iHUVECs connected to each other in the capillary-like structure. Tube area is presented as the average value from three random fields. ** P <0.01 versus the vehicle. ( d , e ) DJ-1 stimulates angiogenesis in vivo . Matrigel plugs containing vehicle, DJ-1 (0.1 or 1 μg) or FGF-2 (0.1 μg) were subcutaneously injected into mice. After 7 days, the matrigel plugs were extracted, fixed, embedded in paraffin, sectioned at 4 μm and immunostained. ( d ) Sections of each matrigel plug were stained by H&E and photographed (X200). The arrow shows blood vessels containing red blood cells. The scale bar represents 10 μm. ( e ) The matrigel plugs were stained with antibody against PECAM (CD31). The scale bar represents 60 μm. n =3 for all groups. All data are expressed as means±s.e.m. Full size image DJ-1 also induced the formation of capillary tubes in iHUVECs, another property related to angiogenesis [1] , [33] . In two-dimensional matrigels, DJ-1 induced the formation of well-organized, capillary-like networks comparable to those induced by FGF-2 ( Fig. 2b ). When the tube area covered by the capillary-like networks was quantified by measuring the lengths of the cells connected to each other in the network, DJ-1 enhanced the area of tube formation about threefold greater than the vehicle control. Similar activities of DJ-1 for promoting migration and tube formation were observed in HUVECs and human microvascular endothelial cells-1 ( Supplementary Figs S5 and S6 ). These results clearly suggest angiogenic properties of DJ-1 in vitro . Next, we performed a matrigel plug assay to investigate if DJ-1 has an angiogenic activity in vivo . Matrigel plugs containing DJ-1 (0.1 or 1 μg), FGF-2 (0.1 μg) or vehicle control were subcutaneously injected into the abdomen of C57BL/six mice. At 7th day after the injection, the matrigel plugs were harvested and examined for blood vessel formation by H&E staining and immunostaining ( Fig. 2d ). Both DJ-1 (1 μg) and FGF-2 significantly stimulated blood vessel formation as compared with vehicle treatment. Blood vessels containing red blood cells were observed in both the DJ-1 (1 μg) and the FGF-2-treated groups ( Fig. 2d ). Blood vessel formation stimulated by DJ-1 treatment was confirmed by immunostaining for CD31, an endothelial marker ( Fig. 2e ). Taken together, these data identify DJ-1 as a novel angiogenic factor that functions both in vivo and in vitro . DJ-1 promotes angiogenesis by activating FGFR-1 To investigate the mechanisms by which DJ-1 displays angiogenic activity in endothelial cells, we asked if DJ-1 could signal through activating receptors for FGF or VEGF. FGFR-1 and VEGF receptor-2 (VEGFR-2) are key receptors that induce angiogenesis in endothelial cells [1] . FGF-2 (20 ng ml −1 ) and VEGF (20 ng ml −1 ) induced the phosphorylation of FGFR-1 and VEGFR-2, respectively, and activated downstream signalling molecules, such as Src kinase, focal adhesion kinase (FAK) and extracellular signal-regulated kinase 1/2 (ERK1/2) [34] , which have been implicated in endothelial cell differentiation ( Fig. 3a ). Importantly, we found that DJ-1 (10 nM) also induced the phosphorylation of FGFR-1 within minutes and activated downstream signalling molecules, such as Src, FAK and ERK1/2. 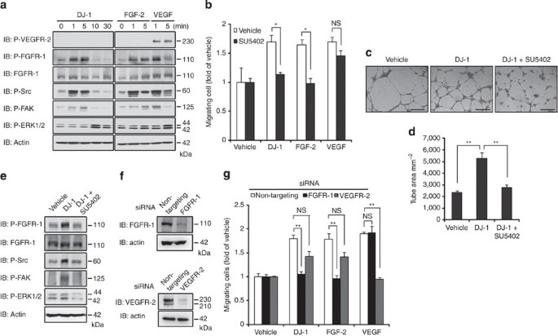Figure 3: DJ-1 induces angiogenesis through FGFR-1 activation. (a) DJ-1 induces FGFR-1 phosphorylation in iHUVECs. Cells were treated with DJ-1 (10 nM), FGF-2 (20 ng ml−1) or VEGF (20 ng ml−1) and phosphorylations of FGFR-1, VEGFR-2, Src, FAK and ERK1/2 were examined. (b) iHUVECs were pretreated with SU5402 (1 μM) for 30 min, and the cells were incubated with DJ-1 (10 nM), FGF-2 (20 ng ml−1) or VEGF (20 ng ml−1) for 6 h to analyse cell migration. NS, not significant and *P<0.05 versus DJ-1 or FGF-2 alone. (c,d) SU5402 (1 μM) abolishes iHUVECs tube formation stimulated by DJ-1. Photographs (X50) were taken at 9 h after treatment with DJ-1 (10 nM), FGF-2 (20 ng ml−1) or vehicle control. The scale bar represents 400 μm. Tube area was also quantified as ind. **P<0.01 versus the vehicle or DJ-1 alone. (e) Shown are representative immunoblots of iHUVECs that were treated with DJ-1 (10 nM) for 5 min in the presence or absence of SU5402 (1 μM). DJ-1-stimulated phosphorylations of FGFR-1, Src, FAK and ERK1/2 were blocked by SU5402 treatment. (f) Knockdown of FGFR-1 or VEGFR-2 by siRNA was confirmed by immunoblot analysis. Cells were harvested at 72 h after transfection with siRNAs (100 nM) for non-targeting, FGFR-1-targeting or VEGFR-2-targeting. (g) The effects of FGFR-1 knockdown on DJ-1-induced iHUVEC migration. iHUVECs were transfected with siRNAs for non-targeting, FGFR-1 or VEGFR-2. At 72 h after transfection, cells were trypsinized and migration activity was investigated. DJ-1 (10 nM), FGF-2 (20 ng ml−1) or VEGF (20 ng ml−1) was treated for 6 h in the cell migration assay. NS, not significant and **P<0.01 versus non-targeting siRNA treatment.n=3 for all groups. All data are expressed as means±s.e.m. Figure 3: DJ-1 induces angiogenesis through FGFR-1 activation. ( a ) DJ-1 induces FGFR-1 phosphorylation in iHUVECs. Cells were treated with DJ-1 (10 nM), FGF-2 (20 ng ml −1 ) or VEGF (20 ng ml −1 ) and phosphorylations of FGFR-1, VEGFR-2, Src, FAK and ERK1/2 were examined. ( b ) iHUVECs were pretreated with SU5402 (1 μM) for 30 min, and the cells were incubated with DJ-1 (10 nM), FGF-2 (20 ng ml −1 ) or VEGF (20 ng ml −1 ) for 6 h to analyse cell migration. NS, not significant and * P <0.05 versus DJ-1 or FGF-2 alone. ( c , d ) SU5402 (1 μM) abolishes iHUVECs tube formation stimulated by DJ-1. Photographs (X50) were taken at 9 h after treatment with DJ-1 (10 nM), FGF-2 (20 ng ml −1 ) or vehicle control. The scale bar represents 400 μm. Tube area was also quantified as in d . ** P <0.01 versus the vehicle or DJ-1 alone. ( e ) Shown are representative immunoblots of iHUVECs that were treated with DJ-1 (10 nM) for 5 min in the presence or absence of SU5402 (1 μM). DJ-1-stimulated phosphorylations of FGFR-1, Src, FAK and ERK1/2 were blocked by SU5402 treatment. ( f ) Knockdown of FGFR-1 or VEGFR-2 by siRNA was confirmed by immunoblot analysis. Cells were harvested at 72 h after transfection with siRNAs (100 nM) for non-targeting, FGFR-1-targeting or VEGFR-2-targeting. ( g ) The effects of FGFR-1 knockdown on DJ-1-induced iHUVEC migration. iHUVECs were transfected with siRNAs for non-targeting, FGFR-1 or VEGFR-2. At 72 h after transfection, cells were trypsinized and migration activity was investigated. DJ-1 (10 nM), FGF-2 (20 ng ml −1 ) or VEGF (20 ng ml −1 ) was treated for 6 h in the cell migration assay. NS, not significant and ** P <0.01 versus non-targeting siRNA treatment. n =3 for all groups. All data are expressed as means±s.e.m. Full size image To determine the possible cross-talk between FGFR-1 signalling and DJ-1-induced angiogenesis, we examined the effects of SU5402, an FGFR-1 antagonist on DJ-1-stimulated iHUVEC migration and capillary tube formation ( Fig. 3b–d ). To our surprise, we found that pretreatment with SU5402 completely blocked the migration of iHUVECs induced by DJ-1. As expected, SU5402 also inhibited FGF-2-induced iHUVEC migration, but not VEGF-induced iHUVEC migration ( Fig. 3b ). The formation of capillary networks induced by DJ-1 was also nearly completely prevented by SU5402 ( Fig. 3c ). In the presence of SU5402, DJ-1 was unable to induce organized structures, and quantification of the tube area confirmed that DJ-1 failed to organize capillary networks when FGFR-1 signalling was disrupted ( Fig. 3d ). Consistent with the lack of effects on migration and network formation, DJ-1 failed to induce the phosphorylations of FGFR-1, Src, FAK and ERK1/2 in the presence of SU5402 ( Fig. 3e ). To further confirm the involvement of FGFR-1 signalling in DJ-1-induced angiogenic activity, we depleted FGFR-1 or VEGFR-2 with a specific small-interfering RNA (siRNA). The efficacy of the FGFR-1 siRNA and VEGFR-2 siRNA was confirmed by immunoblotting ( Fig. 3f ). In a modified Boyden chamber assay, FGFR-1 siRNA completely abrogated iHUVEC migration induced by FGF-2 ( Fig. 3g ). Importantly, we observed that DJ-1 was no longer capable of inducing iHUVEC migration when FGFR-1 was depleted, whereas VEGFR-2 siRNA did not show significant effect on iHUVEC migration stimulated by DJ-1. Collectively, these results indicate that FGFR-1 signalling is required for DJ-1 to induce angiogenic activity in vitro . As we observed activation of FGFR-1 signalling by DJ-1 ( Fig. 3a ), we performed a receptor binding assay by using DJ-1 and iodine-labeled FGF-2 in order to determine whether DJ-1 competes with FGF-2 for the same binding site on FGFR-1 ( Supplementary Fig. S7 ). DJ-1, however, did not compete with FGF-2 for FGFR-1 binding, whereas iodine-labeled FGF-2 competed with unlabelled FGF-2 in a dose-dependent manner. We then examined if DJ-1 has a direct interaction with FGFR-1. To determine the interaction between DJ-1 and FGFR-1, we performed immunoprecipitation of FGFR-1 in the presence or absence of DJ-1. We observed that DJ-1 interacted with FGFR-1 and induced the phosphorylation of FGFR-1 ( Supplementary Fig. S8 ). These results suggest that DJ-1 might activate FGFR-1 by directly interacting with a site that is different from the FGF-2-binding site. DJ-1 stimulates differentiation of hMSCs into osteoblasts Next, we investigated the possible role of DJ-1 in osteogenesis of hMSCs. We found that direct application of exogenous DJ-1 promoted the differentiation and mineralization of osteoblasts in a dose-dependent manner ( Fig. 4a ). Extracellularly applied DJ-1 was sufficient to induce the expression of osteogenic markers, such as ALP, BSP and OCN ( Fig. 4b ). In addition, we found that application of exogenous DJ-1 was capable of inducing VEGF secretion ( Supplementary Fig. S9a ). 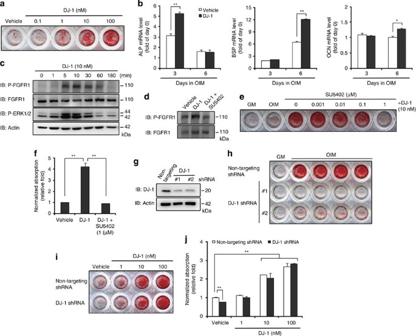Figure 4: DJ-1 stimulates osteoblast differentiation and mineralization of hMSCs. (a) hMSCs were treated with DJ-1 (0.1–100 nM) in osteogenic differentiation condition for 9 days. Osteogenic differentiation was confirmed by alizarin red S staining. (b) Osteogenic marker expression during osteogenesis was confirmed by quantitative reverse transcription-PCR. *P<0.05 and **P<0.01 versus the vehicle. (c) DJ-1 (10 nM) induced phosphorylations of FGFR-1 and ERK1/2 in hMSCs. (d) SU5402 (1 μM) treatment abolished the phosphorylation of FGFR-1 induced by DJ-1. (e) Effect of SU5402 on DJ-1-stimulated osteogenesis was confirmed by alizarin red S staining at 7 days after osteogenesis induction. (f) Quantification of the amount of alizarin red S staining. **P<0.01 versus the vehicle or DJ-1 alone. (g) hMSCs were transfected with non-targeting or two different DJ-1 shRNAs and subjected to immunoblot analysis. (h) Knockdown of DJ-1 by shRNA suppressed osteoblast mineralization, an effect which was confirmed by alizarin red S staining at 12 days after osteogenesis induction. GM indicates growth medium and osteogenesis induction medium (OIM) indicates osteogenesis induction medium. (i) Exogenous DJ-1 rescues osteoblast differentiation in DJ-1 knockdown cells and it was examined by alizarin red S staining at 9 days after osteogenesis induction. (j) Quantification of the amount of alizarin red S staining. **P<0.01 versus the vehicle of non-targeting shRNA treatment.n=3 for all groups. All data are presented as means±s.e.m. Figure 4: DJ-1 stimulates osteoblast differentiation and mineralization of hMSCs. ( a ) hMSCs were treated with DJ-1 (0.1–100 nM) in osteogenic differentiation condition for 9 days. Osteogenic differentiation was confirmed by alizarin red S staining. ( b ) Osteogenic marker expression during osteogenesis was confirmed by quantitative reverse transcription-PCR. * P <0.05 and ** P <0.01 versus the vehicle. ( c ) DJ-1 (10 nM) induced phosphorylations of FGFR-1 and ERK1/2 in hMSCs. ( d ) SU5402 (1 μM) treatment abolished the phosphorylation of FGFR-1 induced by DJ-1. ( e ) Effect of SU5402 on DJ-1-stimulated osteogenesis was confirmed by alizarin red S staining at 7 days after osteogenesis induction. ( f ) Quantification of the amount of alizarin red S staining. ** P <0.01 versus the vehicle or DJ-1 alone. ( g ) hMSCs were transfected with non-targeting or two different DJ-1 shRNAs and subjected to immunoblot analysis. ( h ) Knockdown of DJ-1 by shRNA suppressed osteoblast mineralization, an effect which was confirmed by alizarin red S staining at 12 days after osteogenesis induction. GM indicates growth medium and osteogenesis induction medium (OIM) indicates osteogenesis induction medium. ( i ) Exogenous DJ-1 rescues osteoblast differentiation in DJ-1 knockdown cells and it was examined by alizarin red S staining at 9 days after osteogenesis induction. ( j ) Quantification of the amount of alizarin red S staining. ** P <0.01 versus the vehicle of non-targeting shRNA treatment. n =3 for all groups. All data are presented as means±s.e.m. Full size image We then examined whether DJ-1 stimulated osteogenesis by activating FGFR-1 signalling. As in iHUVECs, DJ-1 induced the activation of FGFR-1 signalling in hMSCs ( Fig. 4c ), an effect which was completely prevented by SU5402 (1 μM) ( Fig. 4d ). Moreover, SU5402 was able to inhibit the mineralization of osteoblasts ( Fig. 4e ). Furthermore, the ability of DJ-1 to induce the expression of osteogenic markers, such as BSP, OCN and bone morphogenic protein 2 (BMP2), was also significantly prevented by SU5402 ( Supplementary Fig. S10 ). In addition, the enhanced expression and secretion of VEGF stimulated by DJ-1 were significantly suppressed in the presence of SU5402 ( Supplementary Fig. S9b,c ). To further confirm the role of DJ-1 in inducing osteogenesis of hMSCs, we applied a specific small hairpin RNA (shRNA) against DJ-1 ( Fig. 4g ) and found that DJ-1 shRNA was able to substantially prevent mineralization of osteoblasts in osteogenic differentiation condition ( Fig. 4h ). On the other hand, treatment of exogenous DJ-1 completely rescued impaired osteogenic differentiation caused by DJ-1 depletion ( Fig. 4i ). In addition, we found that osteogenic activity of FGF-2 was not affected by DJ-1 depletion ( Supplementary Fig. S11 ). Taken together, these results provide convincing evidence that application of extracellular DJ-1 is sufficient to stimulate osteogenesis of hMSCs and that endogenous DJ-1 might be required for mineralization of osteoblasts, but extracellular DJ-1 mainly functions as a strong stimulator of osteogenesis. DJ-1 promotes bone regeneration in a cranial defect model We then examined the possible roles of DJ-1 in the bone healing process by using a rodent model of cranial critical-size defect [35] , [36] , [37] , [38] . Collagen membranes were used as scaffolds and carriers for DJ-1 or FGF-2. Collagen membranes soaked with DJ-1 (1 μg), FGF-2 (0.1 μg) or vehicle control were implanted into the defective areas in the cranial, and then their effects on bone repair were examined by three-dimensional microcomputed tomography (μCT) at 4 weeks after the implantation ( Fig. 5a ). We found that DJ-1 treatment significantly promoted bone repair and that the extent of promotion was comparable to that induced by FGF-2 treatment. New bone formation in the defective site (circled area in Fig. 5a ) was quantified and expressed as a percentage of bone coverage of the total defect area. Histological evaluation of bone repair was also performed by H&E staining ( Fig. 5c ) and immunohistochemistry for antibody against α-SMA (alpha-smooth muscle actin), a marker for vascular muscle ( Fig. 5e ). Again, DJ-1 promoted mature bone formation in the regenerated bone tissue and surrounding soft tissues ( Fig. 5c ). Blood vessels were easily identified in the tissue samples by the positive immunoreactivity with the α-SMA antibody ( Fig. 5e ). The number of blood vessels in the DJ-1-treated group was higher than the vehicle-treated group ( Fig. 5f ). Enhanced bone repair in response to DJ-1 treatment was also noted when observed at 2 weeks ( Supplementary Fig. S12 ). 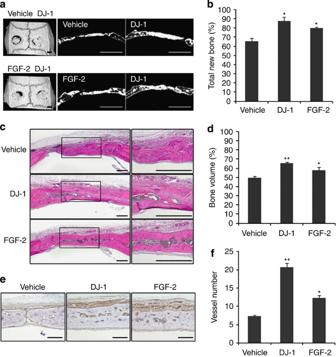Figure 5: DJ-1 promotes bone regeneration in a rat cranial critical-size defect model. (a) Representative μCT images of cranial defects at 4 weeks after surgery. Cranial defect was induced and the defective site was covered with collagen membranes soaked with DJ-1 (1 μg), FGF-2 (0.1 μg) or vehicle control. The scale bar represents 2 mm. (b) Quantification of μCT images of cranial defects at 4 weeks after surgery. Total new bone formation at the defective site is expressed as a percentage of bone coverage relative to the total defective site. *P<0.05 versus the vehicle. (c) At 4 weeks after surgery, defective site sections were stained with H&E and photographed (X40, X100). The scale bar represents 500 μm. (d) Quantification of H&E stained images. Increased bone formation at the defective site in response to application of DJ-1 is shown. Bone volume in the defective site is represented as a percentage of mineralized bone tissue relative to total tissue volume. *P<0.05 and **P<0.01 versus the vehicle. (e) To detect blood vessel formation, defective site sections were immunostained with antibody against α-SMA and photographed (X100). The scale bar represents 200 μm. (f) Quantification of blood vessel in α-SMA-stained images. *P<0.05 and **P<0.01 versus the vehicle.n=8 for all groups (group 1: Vehicle, DJ-1; group 2: DJ-1, FGF-2). All data are presented as means±s.e.m. Figure 5: DJ-1 promotes bone regeneration in a rat cranial critical-size defect model. ( a ) Representative μCT images of cranial defects at 4 weeks after surgery. Cranial defect was induced and the defective site was covered with collagen membranes soaked with DJ-1 (1 μg), FGF-2 (0.1 μg) or vehicle control. The scale bar represents 2 mm. ( b ) Quantification of μCT images of cranial defects at 4 weeks after surgery. Total new bone formation at the defective site is expressed as a percentage of bone coverage relative to the total defective site. * P <0.05 versus the vehicle. ( c ) At 4 weeks after surgery, defective site sections were stained with H&E and photographed (X40, X100). The scale bar represents 500 μm. ( d ) Quantification of H&E stained images. Increased bone formation at the defective site in response to application of DJ-1 is shown. Bone volume in the defective site is represented as a percentage of mineralized bone tissue relative to total tissue volume. * P <0.05 and ** P <0.01 versus the vehicle. ( e ) To detect blood vessel formation, defective site sections were immunostained with antibody against α-SMA and photographed (X100). The scale bar represents 200 μm. ( f ) Quantification of blood vessel in α-SMA-stained images. * P <0.05 and ** P <0.01 versus the vehicle. n =8 for all groups (group 1: Vehicle, DJ-1; group 2: DJ-1, FGF-2). All data are presented as means±s.e.m. Full size image To investigate whether FGFR-1 activation is crucial for DJ-1-stimulated bone regeneration in vivo as observed in vitro ( Figs 3 and 4 ), we examined the effects of SU5402 (15 μg) and found that SU5402 treatment completely prevented bone regeneration induced by DJ-1 ( Supplementary Fig. S13a,b ). Similarly, inductive blood vessel formation induced by DJ-1 was also blocked by SU5402 treatment ( Supplementary Fig. S13c ). These results show that FGFR-1 activation is required for the in vivo functions of DJ-1 to promote bone regeneration and blood vessel formation. DJ-1 -deficient mice show impaired bone regeneration To further investigate the in vivo role of DJ-1 in bone regeneration, we performed surgery to induce cranial defects (4 mm in diameter) in DJ-1 −/− mice and wild-type (6-weeks-old). After 3 weeks, the general aspects of bone regeneration were observed by trichrome stained sections ( Fig. 6a ). In both wild-type and DJ-1 −/− mice, new bone formation from bone margins was observed, and the healing was proceeded mainly through a thin fibrous connective tissue. Notably, DJ-1 −/− mice (7.73±1.49%) showed defects in new bone formation as compared with wild-type (12.87±3.05%). In both DJ-1 −/− mice and wild-type, the newly formed bone, however, was not detected in μCT image because of insufficient maturation of bone matrix. Most of the newly formed bone tissues observed at the marginal areas revealed immature woven bones surrounded by thin lamellar plates. Moreover, in DJ-1 −/− mice (0.61±0.15%), the mineral apposition rate (MAR) at tibial cortical plate was also reduced compared with wild-type (1.19±0.14%), suggestive of impaired bone formation ( Fig. 6c ). Similarly, impaired blood vessel formation in the cranial defective site was observed in DJ-1 −/− mice as compared with wild-type ( Supplementary Fig. S14 ). Taken together, these results show that DJ-1 is an important regulator of bone regeneration in vivo . 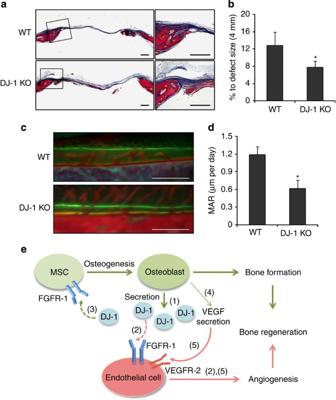Figure 6:DJ-1-deficient mice show reduced bone regeneration in a cranial critical-size defect model. (a) Surgery was performed to induce cranial defects in wild-type (WT) andDJ-1−/−mice (DJ-1 KO). After 3 weeks, bone defective site sections were examined by trichrome staining and photographed (X40, X100). The scale bar represents 300 μm. (b) Efficiency of bone regeneration was evaluated by measuring of the linear ingrowth of new bones from defective margins and expressed as a percentage to the total defective size. *P<0.05 versus WT. (c) Double fluorescent labels were shown at tibial cortical plate and photographed (X200). The scale bar represents 300 μm. (d) Distance between the two fluorescent labels was measured to represent the MAR (μm per day) of new bone formation. *P<0.05 versus MAR of WT.n=3 for all groups. All data are expressed as means±s.e.m. (e) Proposed mechanism for a role of DJ-1 in bone regeneration. First, DJ-1 is secreted during MSC osteogenesis. Second, secreted DJ-1 induces the migration and differentiation of endothelial cells to form functional blood vessels via activation of FGFR-1 signalling. Third, DJ-1 stimulates the osteogenesis of MSCs via FGFR-1 activation and, fourth, DJ-1 also enhances VEGF secretion during osteogenesis. Fifth, upregulation of both DJ-1 and VEGF during osteogenesis can accelerate angiogenesis at the fracture site and enhance bone regeneration. Figure 6: DJ-1 -deficient mice show reduced bone regeneration in a cranial critical-size defect model. ( a ) Surgery was performed to induce cranial defects in wild-type (WT) and DJ-1 −/− mice (DJ-1 KO). After 3 weeks, bone defective site sections were examined by trichrome staining and photographed (X40, X100). The scale bar represents 300 μm. ( b ) Efficiency of bone regeneration was evaluated by measuring of the linear ingrowth of new bones from defective margins and expressed as a percentage to the total defective size. * P <0.05 versus WT. ( c ) Double fluorescent labels were shown at tibial cortical plate and photographed (X200). The scale bar represents 300 μm. ( d ) Distance between the two fluorescent labels was measured to represent the MAR (μm per day) of new bone formation. * P <0.05 versus MAR of WT. n =3 for all groups. All data are expressed as means±s.e.m. ( e ) Proposed mechanism for a role of DJ-1 in bone regeneration. First, DJ-1 is secreted during MSC osteogenesis. Second, secreted DJ-1 induces the migration and differentiation of endothelial cells to form functional blood vessels via activation of FGFR-1 signalling. Third, DJ-1 stimulates the osteogenesis of MSCs via FGFR-1 activation and, fourth, DJ-1 also enhances VEGF secretion during osteogenesis. Fifth, upregulation of both DJ-1 and VEGF during osteogenesis can accelerate angiogenesis at the fracture site and enhance bone regeneration. Full size image Through an unbiased search for molecules that have angiogenic activity, here we identify DJ-1 as a novel factor that promotes angiogenesis and stimulates osteogenesis ( Fig. 6e ). We have found that DJ-1 secretion is significantly enhanced during hMSC osteogenesis and that DJ-1 stimulates blood vessel formation in endothelial cells through the activation of FGFR-1 signalling. Moreover, direct application of DJ-1 in the medium was sufficient to stimulate the differentiation of hMSCs into osteoblasts by inducing FGFR-1 activation and VEGF secretion from osteoblasts. These activities of DJ-1 led to enhanced bone regeneration in vivo by stimulating angiogenesis and bone formation during bone fracture healing process. Together, our findings suggest DJ-1 as a novel angiogenic factor and an activator of osteogenesis that mediates the communication between osteoblasts and endothelial cells during bone regeneration. Bone regeneration is a complicated process that requires interactions among diverse cell-types. During bone regeneration, skeletal vascularization of the fracture site is crucial and the interaction between bone-forming osteoblasts and endothelial cells is of particular importance. This cross-talk is likely mediated by secretory molecules that function in an autocrine and/or paracrine fashion, but the identities of the molecules that mediate the interaction have not been fully defined. Here we identify DJ-1 as a novel mediator of cross-talk between osteoblasts and endothelial cells through the proteomic analysis of osteoblast CM. As we found that osteoblast CM included a variety of proteins with osteogenic or angiogenic activity, as previously described, it is also possible that DJ-1 might participate in bone regeneration together with or by regulating these secretory molecules of osteoblasts. VEGF and FGF-2 are well-known to stimulate osteoblast differentiation [39] , [40] . VEGF promotes osteogenic differentiation in vitro and local application of VEGF in vivo enhances bone healing, whereas inhibition of VEGF activity impairs fracture healing [41] , [42] . Similarly, FGF-2 has been previously identified as a major player in angiogenesis and skeletal development [43] . FGF-2 treatment stimulates bone formation in vitro and depletion of FGF-2 gene suppresses osteogenic differentiation of MSCs [44] . In addition, expression of FGFs and their receptors are known to be elevated during fracture healing [19] and local application of recombinant human FGF-2 accelerates healing of tibial shaft fractures in human [45] . Here we show that application of exogenous DJ-1 is sufficient to induce both angiogenesis and osteogenesis in vitro and that VEGF secretion is markedly increased in response to DJ-1 treatment during osteogenesis ( Supplementary Fig. S9a ). Moreover, administration of DJ-1 enhances bone regeneration in vivo by stimulating the formation of blood vessels and new bones in a rodent model of cranial critical-size defect ( Fig. 5 ). Given that VEGF secretion from osteoblasts is upregulated by application of DJ-1 ( Supplementary Fig. S9a ), it is possible that DJ-1 enhances angiogenesis and bone formation by activating both FGFR-1 and VEGFR-2 signalling. Our results show that depletion of DJ-1 in hMSCs suppressed their differentiation into osteoblasts and mineralization as well ( Fig. 4h ). Together with the fact that DJ-1 secretion was inhibited during osteogenesis when mineralization was blocked ( Fig. 1e ), these results suggest that DJ-1 might act in an autocrine/paracrine fashion during osteoblast mineralization. Moreover, as the expression level of DJ-1 did not represent the enhanced secretion of DJ-1 during osteogenesis ( Supplementary Fig. S3 ), it is supposed that mineralization of osteoblasts induces the translocation of DJ-1 to the extracellular region and that secretory DJ-1 might stimulate further differentiation into mature osteoblasts. In experimental condition, bone regeneration was impaired in DJ-1 -knockout mice ( Fig. 6 ). Given that DJ-1 -deficient mice do not display obvious defects in the formation of bones or vessels during development, DJ-1 might not be a major factor for regulating such processes under normal conditions. It is, however, possible that DJ-1 is activated and regulates angiogenesis and osteogenesis under particular physiological conditions, such as bone fracture, a process which requires extensive bone regeneration. Further study will be needed to elucidate the conditions that induce the secretion and activation of DJ-1. Moreover, verification of phenotype in DJ-1 -knockout mice by using alternative bone fracture model, such as a long bone fracture assay [46] , would further support the in vivo function of DJ-1 in bone regeneration. As MAR was reduced in the tibia of DJ-1 -knockout mice ( Fig. 6c ), impaired and delayed bone healing might be shown in DJ-1 -knockout mice in response to other bone fracture. DJ-1 is thought to be a causative gene for PARK7 -linked early-onset Parkinson’s Disease [23] . Although the precise roles of DJ-1 remains to be defined, several studies have suggested that DJ-1 functions intracellularly as a molecular chaperon [24] , as a transcriptional regulator [47] and as a pro-survival factor [25] , [26] . Interestingly, there have been studies reporting the presence of DJ-1 in serum [27] , [28] and some suggestions have been made regarding the mechanisms that might mediate the secretion of DJ-1 into the medium [48] . The extracellular function, however, of the secreted DJ-1 has remained ambiguous. This study assigns novel extracellular functions to DJ-1 and demonstrates its role as an activator of angiogenesis and osteogenesis. We also suggest that these functions are mediated by activating FGFR-1 signalling on the basis of our observation that DJ-1 induced the phosphorylation of FGFR-1, as well as downstream signalling molecules in endothelial cells and hMSCs and that knockdown or inhibition of FGFR-1 signalling suppressed DJ-1-stimulated angiogenic and osteogenic activities. As DJ-1 did not compete with FGF-2 for binding to FGFR-1, but DJ-1 had a direct interaction with FGFR-1 ( Supplementary Figs S7 and S8 ), it is supposed that DJ-1 functions as a ligand for FGFR-1 by binding to a site distinct from the FGF-2-interaction site. It is, however, also plausible that DJ-1 activates FGFR-1 through an interaction with co-receptor or modulator of FGFR-1, which forms complex with FGFR-1 and might regulate the activation of FGFR-1 [4] , [49] . Notably, application of extracellular DJ-1 caused a marked elevation in the mRNA levels of BSP and OCN, an effect which was substantially, but only partially blocked by SU5402 ( Supplementary Fig. S10 ). By contrast, DJ-1-induced upregulation of BMP2 mRNA ( Supplementary Fig. S10 ), as well as the formation of capillary network ( Fig. 3c ) and cell migration ( Fig. 3b ) were completely blocked by antagonizing FGFR-1 signalling. These results suggest that some signals induced by DJ-1 are mediated by FGFR-1 signalling, but other signals might require additional signalling. In addition, our results suggest the possibilities that DJ-1 and FGFR-1 act together in same type of cells or interact with each other in two different types of cells. Our data show that DJ-1 secretion is upregulated during osteogenesis and that secretory DJ-1 might function as an activator of osteogenesis and angiogenesis through FGFR-1 signalling. Accordingly, DJ-1 and FGFR-1 might act together in MSCs and/or osteoblasts when DJ-1 function as an osteogenic activator. On the other hand, when DJ-1 functions as an angiogenic factor, secretory DJ-1 from osteoblasts might interact with FGFR-1 in endothelial cells. Although the detailed molecular mechanisms by which DJ-1 activates FGFR-1 signalling or possibly other signalling need further investigation, our study clearly reveals previously undefined extracellular roles of DJ-1. In conclusion, our study adds DJ-1 to the limited list of exogenous factors that induce osteogenesis and angiogenesis, both of which properties are essential for bone regeneration. Our work suggests that DJ-1 in vivo might have a therapeutic potential for promoting vascular supply and bone fracture healing. Furthermore, given that there is limited therapy for the bone fracture healing, combination treatment of DJ-1 with angiogenic factors, such as VEGF and FGF-2 or osteogenic factors, such as BMP2 and BMP4 [36] , [50] , may provide a new therapeutic strategy to improve bone regeneration. Cells and culture conditions hMSCs were purchased from Cambrex (Lonza, Walkersville, MD) and maintained in DMEM (Lonza) supplemented with 10% FBS (Gibco BRL, Grand Island, NY), 100 units ml −1 penicillin and 0.1 mg ml −1 streptomycin (Gibco BRL). Human papilloma virus immortalized HUVECs (iHUVECs, kindly provided by Dr Ashley Moses, Oregon Health & Sciences University) were maintained in M199 supplemented with 10% FBS (Lonza), 5 mM L -glutamine (Gibco BRL), endothelial cell growth supplement (ECGS, BD Biosciences, Bedford, MA), 100 units ml −1 penicillin and 0.1 mg ml −1 streptomycin. The cells were grown at 37 °C under a humidified atmosphere with 5% CO 2 . Cells for all experiments were used at passages 6–10. Osteogenic differentiation of hMSCs and alizarin red S staining hMSCs were plated 3 × 10 5 per in 6-well plates or 1 × 10 4 per in 96-well plates. After 2 days, hMSCs were cultured in DMEM supplemented with 10% FBS, 10 mM β-glycerophosphate (USB Corp, Cleveland, OH), 50 μM ascorbate-2-phosphate (Sigma-Aldrich, St Louis, MO), 100 nM dexamethasone (Sigma-Aldrich), 100 units ml −1 penicillin and 0.1 mg ml −1 streptomycin. Osteoblast differentiation of hMSCs was confirmed by alizarin red S staining. For staining, differentiated cells were fixed in 4% paraformaldehyde for 20 min, washed two times with PBS, and then stained with 1% alizarin red solution (Sigma-Aldrich) for 20 min. Cells were then washed five times with distilled water and examined for the presence of calcium deposits. Mineralization was quantified as previously described [51] . Detection of DJ-1 secretion Concentration of DJ-1 in the medium was measured by using a Human DJ-1 ELISA kit (CircuLex Co, Japan) according to the manufacturer’s protocol. Cell migration assay Cell migration was measured in a modified Boyden chemotaxis chamber (NeuroProbe Inc, Gaithersburg, MD). Polycarbonated membranes with 8 μm pores were coated with 20 μg human placenta collagen (Sigma-Aldrich) and dried. M199 medium containing vehicle or test compounds was placed in the bottom wells of the chamber. Cells were trypsinized and washed, and then resuspended in M199. The upper chamber was loaded with 1 × 10 4 cells. The chemotaxis chambers were incubated at 37 °C for 6 h. After incubation, non-migrating cells were removed from the top side of the filter, and migrated cells were stained with Hoechst dye (Sigma-Aldrich). Five randomly chosen fields (X100) of each sample were photographed and counted. Endothelial cell capillary tube formation assay iHUVECs (1 × 10 5 cells per well) were plated into 48-well plates coated with growth factor-reduced matrigel (BD Biosciences) and incubated for 9 h at 37 °C in serum-free M199 in the presence of test compounds as indicated. Three random areas for each sample were photographed. Using the Scion Image Programme, total tube areas were measured in mm 2 . All images were visualized by using a Zeiss Axiovert 135 microscope equipped with an Olympus DP71 camera. Matrigel plug assay and immunostaining The matrigel plug assay was performed as previously described [52] . C57BL/six mice (male, 6 weeks, three mice per group) were subcutaneously injected in the abdomen with 0.5 ml of growth factor-reduced matrigel plugs containing test compounds supplemented with 10 units of heparin to promote angiogenesis. The mice were euthanized at 7th day after implantation, and then matrigel plugs were harvested. The plugs were fixed in 4% paraformaldehyde and embedded in paraffin. Cross-sections of paraffin-embedded matrigel were stained with hematoxylin and eosin (H&E) and images were visualized using an Olympus BX51 microscope equipped with an UPlanFL XN100/1.30 oil objective lens. For vessel immunostaining, anti-CD31 antibody (1:1,000, Santa Cruz Biotechnology, Santa Cruz, CA) was used. All images were visualized using an FV1000 Olympus confocal microscope equipped with an UPlanSApo X40/0.75 objective lens and acquired by using FV1000-ASW 1.5 software. Animal study protocols were approved by the Institutional Animal Care and Use Committee at Pohang University of Science and Technology. Knockdown of FGFR-1 and VEGFR-2 siRNA duplexes directed against FGFR-1 (5′-AAGAAATTGCATGCAGTGCCG-3′ [53] ), VEGFR-2 (5′-GGAATTGACAAGACAGCAA-3′) and non-targeting siRNA duplexes (5′-TTCTCCGAACGTGTCACGT-3′) were synthesized by GenePharma (Shanghai, China). iHUVECs were transfected with siRNA (100 nM) for non-targeting, FGFR-1-targeting or VEGFR-2-targeting using lipofectamine (Invitrogen) under serum-free conditions according to the manufacturer’s instructions. At 4 h after transfection, the cells were washed and supplemented with fresh medium containing 10% foetal bovine serum. Cells were incubated for 72 h before use. Knockdown of DJ-1 Lentiviral shRNA expression plasmids for non-targeting and human DJ-1 ( PARK7 ) were purchased from Sigma-Aldrich (St Louis, MO). Non-targeting shRNA plasmid (SHC002: 5′-CCGGCAACAAGATGAAGAGCACCAACTCGAGTTGGTGCTCTTCATCTTGTTGTTTTT-3′) and human PARK7 -targeting shRNA plasmids (#1: NM_007262.3-583s1c1, 5′-CCGGGCAATTGTTGAAGCCCTGAATCTCGAGATTCAGGGCTTCAACAATTGCTTTTT-3′, #2: NM_007262.3-506s1c1, 5′-CCGGACTCTGAGAATCGTGTGGAAACTCGAGTTTCCACACGATTCTCAGAGTTTTTT-3′). For lentivirus transduction, 293T cells were transfected with 10 μg vector, 5 μg G protein of the vesicular stomatitis virus (VSV-G) and 7.5 μg Δ 8.9 in 15 cm 2 dish. Viral supernatant was harvested at 72 h after transfection and hMSCs were transfected with viral supernatant using lipofectamine (Invitrogen). Cells were cultured in the puromycin-containing medium (2 μg ml −1 ) for 2 days to select shRNA-transfected cells. After selection, cells were plated to be cultured. Bone regeneration in a rat cranial defect model In vivo bone regeneration activity of DJ-1 was examined as previously described [35] with minor modifications. Lewis rats (male, 12 weeks) were anesthetized. Using aseptic routines, a 15-mm incision was made through the skin over the cranium and periosteum and then full-thickness flaps were raised. Under sterile saline irrigation, a circular 9 mm diameter defect was created by a trephine bur in the rat cranium (rat cranium critical defect size: 8 mm). After the full-thickness of the cranial bone was removed, collagen membranes (Zimmer Dental) with test compounds were immediately placed in the defect. After 2–4 weeks, the defective sites were analysed with a three-dimensional microcomputed (μCT) system (x-eye MCT series, SEC Co, Republic of Korea). Tissue sections of the defective site were stained by H&E or α-SMA (Cell Marque, Rocklin, CA) antibody. All images were visualized using an Olympus BH2 microscope equipped with an Olympus DP50 digital camera. Bone volume was expressed as a percentage of mineralized bone tissue relative to the total tissue volume and was measured by an iSolution DT analysis system (iMTechnolog, Daejeon, Republic of Korea). Blood vessel analyses were also performed by iSolution DT. Animal study protocols were approved by the Institutional Animal Care and Use Committee at Kyungpook National University. DJ-1 -knockout mice DJ-1 -knockout mice on a C57BL/six background [54] were kindly provided by Tak W. Mak (University of Toronto, Toronto, ON, Canada). Bone regeneration in DJ-1 -knockout mice Wild-type and DJ-1 −/− mice (male, 6 weeks, three mice of each group) were anesthetized. The skin over the cranium was shaved and 0.5 cm midline sagittal incision was made to expose bone. Using a 4-mm external diameter dental trephine bur, one transosseous defect was created in the parietal calvarium lateral to the sagittal suture under constant saline irrigation. And then the defective site was covered by layer suture of perisosteum and skin with 5/0 absorbable monocryl suture (Ethicon, NJ). After surgery, the animals were injected subcutaneously with gentamicin antibiotic for 3 days. In addition, oxytetracycline (0.3 ml kg −1 ) was injected intramuscularly twice in a 12-day-interval for MAR evaluation. Animals were killed at 3 weeks after surgery. Block sections, including the surgical sites, were removed and fixed in 10% neutral-buffered formalin. Specimens were decalcified in 10% EDTA and embedded in paraffin. Five micrometre thickness coronal sections were cut and stained with trichrome. In addition, the tibia from each animal was prepared for resin embedded grind sections of 30 μm thickness. Histomorphometric data were evaluated using an analysis programme ( i MT image analysis software). For MAR analysis, the width of the newly mineralized bone layer at the cortex of tibia, expressed in units of microns per day, was determined by measuring the distance between two parallel fluorescent labels (tetracycline stained lines, detected at 390 nm). All images were obtained using Olympus BH2 microscope equipped with an Olympus DP50 digital camera. Statistical analysis The data were analysed using Student’s t -test. P <0.05 and P <0.01 were considered significant. All of the experiments presented in the present study were repeated at least three times. Additional information about cell culture, preparation of CM, reverse-phase high-performance liquid chromatography, tryptic digestion, electrospray ionization liquid chromatography-mass spectrometry, DJ-1 purification, human microvascular endothelial cells-1 image, receptor binding competition assay, immunoprecipitation, detection of VEGF concentration, visualization of vessel formation, RNA extraction, quantitative reverse transcription-PCR, immunoblotting and general reagents can be found in the Supplementary Information . How to cite this article: Kim J.-M. et al. DJ-1 promotes angiogenesis and osteogenesis by activating FGF receptor-1 signaling. Nat. Commun. 3:1297 doi: 10.1038/ncomms2313 (2012).